The deubiquitinating enzyme CYLD controls apical docking of basal bodies in ciliated epithelial cells CYLD is a tumour suppressor gene mutated in familial cylindromatosis, a genetic disorder leading to the development of skin appendage tumours. It encodes a deubiquitinating enzyme that removes Lys63- or linear-linked ubiquitin chains. CYLD was shown to regulate cell proliferation, cell survival and inflammatory responses, through various signalling pathways. Here we show that CYLD localizes at centrosomes and basal bodies via interaction with the centrosomal protein CAP350 and demonstrate that CYLD must be both at the centrosome and catalytically active to promote ciliogenesis independently of NF-κB. In transgenic mice engineered to mimic the smallest truncation found in cylindromatosis patients, CYLD interaction with CAP350 is lost disrupting CYLD centrosome localization, which results in cilia formation defects due to impairment of basal body migration and docking. These results point to an undiscovered regulation of ciliogenesis by Lys63 ubiquitination and provide new perspectives regarding CYLD function that should be considered in the context of cylindromatosis. Centrioles are conserved microtubule-based organelles displaying structural asymmetry, with the mother centriole bearing two sets of appendages at its distal end. In resting cells, the mother centriole can turn into a so-called basal body and dock to the plasma membrane through the distal appendages, to complete primary cilia formation [1] . In addition to these primary cilia, multiple motile cilia are present in some mammalian epithelia (for example, brain ventricles, respiratory tract and fallopian tubes). In contrast to cycling cells, these multiciliated cells have the ability to assemble hundreds of centrioles that anchor to the plasma membrane and grow cilia [2] . In all cases, ciliogenesis is a multistep process that includes basal body assembly, maturation and migration, transition zone formation, docking to the cell surface and further axonemal extension, which requires intraflagellar transport [3] . Primary cilia are considered as cell antennas that receive extracellular signals and transmit them to the cell bodies, thus coordinating cell growth, polarity and differentiation [4] , [5] . Among their role in sensing the environment, cilia are required to mediate several signal transduction pathways [6] . Therefore, any defects in this organelle lead to a wide range of developmental disorders and diseases grouped under the term ‘ciliopathies’ [1] . Among the numerous centrosomal proteins, CAP350 serves as a platform to anchor several proteins to the centrosome. FOP (FGFR1 oncogene partner) localization at the centrosome depends on its association with CAP350 and is required to recruit EB1 at the centrosome [7] . The complex CAP350/FOP was shown to be required for microtubule anchoring to the centrosome. In addition, as a microtubule binding protein CAP350 stabilizes the microtubule network [8] as well as the microtubules of the centriolar barrel [9] , allowing the maintenance of a continuous pericentrosomal golgi ribbon [8] . Interestingly, removal of EB1 from the centrosome by expression of a carboxy-terminal fragment of CAP350 as well as depletion of FOP inhibits primary cilia formation [10] . CYLD was originally identified as a gene mutated in familial cylindromatosis, a genetic condition that predisposes patients to the development of skin appendages tumours, referred to as cylindromas. Patients with cylindromatosis carry heterozygous germ-line mutations in the CYLD gene [11] . During their life, some cells undergo a loss of heterozygosity with the disappearance of the wild-type (WT) CYLD allele. The remaining mutated allele leads to the expression of a truncated protein, thus resulting in the development of cylindromas. Therefore, this mode of tumour formation defines CYLD as a tumour suppressor. The CYLD gene encodes a deubiquitinating (DUB) enzyme, which removes lysine 63-linked polyubiquitin chains (K63-linked ubiquitin) as well as linear chains from target proteins [12] . Interestingly, most of the mutations of CYLD found in human cylindromas are predicted to cause C-terminal truncations and catalytic inactivation of the DUB domain. The CYLD protein was shown to regulate cell survival and inflammatory responses mainly through inhibiting nuclear factor-κB (NF-κB) and mitogen-activated protein (MAP) kinase signalling [13] , [14] . In addition, CYLD was also shown to negatively regulate the Wnt/β-catenin signalling pathway by removing K63-linked ubiquitin of Dishevelled (Dvl) [15] , and more recently CYLD was found to interact with the centrosomal protein CEP192 (ref. 16 ), which plays a critical role in centrosome biogenesis [17] . The tumour suppressing function of CYLD has been studied, in vivo , using Cyld knockout (KO) mice. Surprisingly, these mice do not spontaneously develop tumours but their skin is more sensitive to tumorigenic chemicals compared with WT mice [18] . Intriguingly, transgenic mice, which carry a complete deletion of the DUB domain ( Cyld Δ9/Δ9 ) die perinatally from respiratory dysfunction and exhibit immature lungs characterized by hyperplasic mesenchyme [19] . The striking difference between those two phenotypes led us to use a knockin mouse model engineered to recapitulate more closely the smallest truncation found in patients by expressing a truncated CYLD protein lacking the last 24 C-terminal amino acids of its catalytic domain ( Cyld Δ932 ). To further characterize how CYLD may contribute to cylindromatosis onset, we highlight the interaction between CYLD and the centrosomal CAP350 protein, which leads to CYLD localization to the centrosome. In addition, we demonstrate that Cyld Δ932 mice show impaired apical migration and docking of basal bodies in multiciliated cells with a concomitant loss of CYLD centrosomal localization and CAP350 interaction. To understand the mechanism by which CYLD impairs basal body migration/docking, we expressed several constructs of the protein and show that CYLD overexpression in the cytosol prevents primary cilia formation, while its specific expression at the centrosome leads to primary cilia formation. Conversely, expression of the catalytically inactive CYLD at the centrosome abolishes ciliogenesis. This demonstrates that both centrosome localization and CYLD DUB activity are required for cilia formation. Finally, we demonstrate by inhibiting the NF-κB pathway that catalytically inactive CYLD abolishes ciliogenesis in an NF-κB-independent manner. Altogether, these results point to an unravelled role of Lysine 63 ubiquitination in ciliogenesis. CYLD interacts with CAP350 at the centrosome/basal bodies We identified CYLD as a potential interacting partner of CAP350, by performing immunoprecipitation directed against CAP350 followed by mass spectrometry analysis. Eleven peptides were found in the 110-kDa band that matched sequences throughout the tumour suppressor protein CYLD ( Fig. 1a and Supplementary Fig. 1 ). We confirmed the presence of CYLD in the CAP350 immunoprecipitate using a monoclonal antibody directed against the catalytic domain of CYLD ( Fig. 1b ), thus establishing CAP350/CYLD interaction. To further map the interacting domains of CAP350 and CYLD, we transfected Myc-tagged DNA constructs encoding various portions of CAP350 with full-length Flag-tagged CYLD into HEK 293T cells and performed immunoprecipitation with an anti-Flag antibody. The CYLD interacting domain was mapped to the C-terminal domain of CAP350 ( Fig. 1c ). As full-length CAP350 is insoluble, we overexpressed the CAP350 C-terminal domain with either a CYLD ΔN (AA394-956) or CYLD ΔC (AA1-585) construct. We found that the CAP350 C-terminal domain interacts with a CYLD ΔN (AA394-956) protein but not with the CYLD ΔC (AA1-585) protein, suggesting that it interacts with the DUB domain of CYLD ( Fig. 1d ). In addition, cells co-expressing both proteins show a co-localization of CAP350-GFP and CYLD-Flag to the centrosome and to the microtubules ( Supplementary Fig. 2a ). Such localization has already been observed for CAP350 overexpression alone, as previously described [8] , while CYLD-Flag expressed alone was present in the cytosolic fraction ( Supplementary Fig. 2b ). These results suggest that CAP350 directs CYLD localization to perform specific functions in cells. 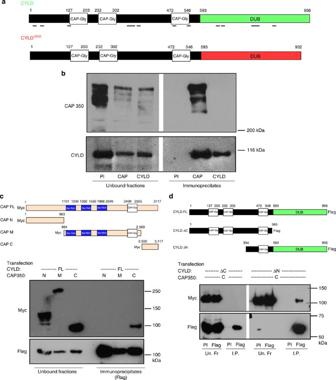Figure 1: CYLD interaction with CAP350. (a) Schematic representation of the CYLD protein with the three CAP-Gly domains and the catalytic DUB domain (593–956). The locations of the 11 peptides found by mass spectrometry are underlined. In the lower panel, representation of the truncated protein expressed inCyldΔ932mice, which lacks the last 24AA of the the DUB domain. (b) IP experiments were performed on RPE1 cells using pre-immune (PI, as control), polyclonal anti-CAP350 (CAP), or monoclonal anti-CYLD (CYLD) IgGs. The immunoprecipitated proteins and non-associated components are referred to as ‘Immunoprecipitates’ and ‘unbound fraction’, respectively. IP products were analysed by WB analysis using antibodies directed against CAP350 and CYLD (polyclonal) as indicated. CAP, CAP350. (c) Full-length CYLD-Flag and three CAP350 fragments as schematized above were expressed in HEK293. CYLD-Flag immunoprecipitates the C-terminal domain of CAP350. (d) CAP350 C-terminal domain and either CYLD ΔC (1–585) and CYLD ΔN (394–956) were expressed in HEK293. CYLD ΔN immunoprecipates the C-terminal domain of CAP350. Un.Fr, unbound fractions; IP, Immunoprecipitates. Figure 1: CYLD interaction with CAP350. ( a ) Schematic representation of the CYLD protein with the three CAP-Gly domains and the catalytic DUB domain (593–956). The locations of the 11 peptides found by mass spectrometry are underlined. In the lower panel, representation of the truncated protein expressed in Cyld Δ932 mice, which lacks the last 24AA of the the DUB domain. ( b ) IP experiments were performed on RPE1 cells using pre-immune (PI, as control), polyclonal anti-CAP350 (CAP), or monoclonal anti-CYLD (CYLD) IgGs. The immunoprecipitated proteins and non-associated components are referred to as ‘Immunoprecipitates’ and ‘unbound fraction’, respectively. IP products were analysed by WB analysis using antibodies directed against CAP350 and CYLD (polyclonal) as indicated. CAP, CAP350. ( c ) Full-length CYLD-Flag and three CAP350 fragments as schematized above were expressed in HEK293. CYLD-Flag immunoprecipitates the C-terminal domain of CAP350. ( d ) CAP350 C-terminal domain and either CYLD ΔC (1–585) and CYLD ΔN (394–956) were expressed in HEK293. CYLD ΔN immunoprecipates the C-terminal domain of CAP350. Un.Fr, unbound fractions; IP, Immunoprecipitates. Full size image CYLD localizes to the centrosome and basal bodies This CAP350/CYLD interaction prompted us to investigate the localization of endogenous CYLD. To that end, we generated and affinity purified an antibody directed against CYLD (CYLD 089). Staining with this antibody showed that CYLD is enriched at the centrosome throughout the cell cycle ( Fig. 2a,b ). In addition, a faint labelling of the nucleus was observed in interphase cells. Such a nuclear staining has previously been observed for several ciliary or centrosomal proteins [20] . During metaphase, CYLD was detected along some spindle microtubules and at the spindle poles ( Fig. 2b ), reminiscent of CAP350 staining [8] . To further ascertain this centrosomal localization, we used a biochemical approach. Western blot (WB) analysis with two antibodies against CYLD identified a major band at 110 kDa, which was specifically enriched in the centrosomal fraction of KE37 cells but also weakly detected in Triton X-100-soluble and -insoluble fractions ( Fig. 2c ). Consistent with these observations, purified centrosomes were strongly labelled by CYLD antibodies ( Fig. 2d ). We conclude that CYLD is a centrosomal protein. 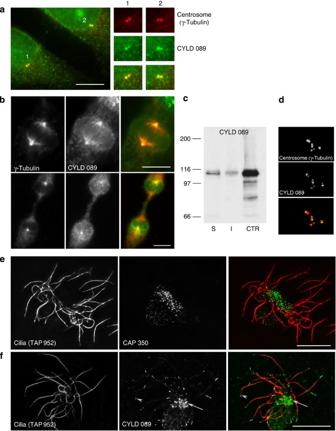Figure 2: CYLD localizes to the centrosome and basal bodies. (a) Double labelling of RPE1 cells with polyclonal affinity-purified CYLD antibody (CYLD 089) and the monoclonal γ-tubulin antibody GTU88, which recognizes the centrosome. (b) CYLD staining in RPE1 during metaphase (upper panel) and telophase (lower panel) with antibodies directed against CYLD and γ-tubulin. During metaphase, CYLD remains localized to the centrosome but is also present along the spindle as previously described for CAP350 (ref.8). During telophase, CYLD antibodies label the centrosome and some dots around it. Staining of the midbody and the central spindle was never observed. (c) WB analysis of CYLD in Triton X-100-soluble (S) and insoluble (I) protein fractions and a highly enriched centrosomal fraction (CTR) from KE37 cells. (d) Immunostaining of isolated centrosomes with polyclonal affinity-purified CYLD antibody (CYLD089) and CTR453. (e) Deconvoluted images of cultured ependymal cells stained with antibodies against CAP350 and TAP 952. (f) Deconvoluted images of cultured ependymal cells stained with antibodies against CYLD and TAP 952. Note that CYLD stained not only basal bodies but also cilia tips. Scale bars, 10 μm. Figure 2: CYLD localizes to the centrosome and basal bodies. ( a ) Double labelling of RPE1 cells with polyclonal affinity-purified CYLD antibody (CYLD 089) and the monoclonal γ-tubulin antibody GTU88, which recognizes the centrosome. ( b ) CYLD staining in RPE1 during metaphase (upper panel) and telophase (lower panel) with antibodies directed against CYLD and γ-tubulin. During metaphase, CYLD remains localized to the centrosome but is also present along the spindle as previously described for CAP350 (ref. 8 ). During telophase, CYLD antibodies label the centrosome and some dots around it. Staining of the midbody and the central spindle was never observed. ( c ) WB analysis of CYLD in Triton X-100-soluble (S) and insoluble (I) protein fractions and a highly enriched centrosomal fraction (CTR) from KE37 cells. ( d ) Immunostaining of isolated centrosomes with polyclonal affinity-purified CYLD antibody (CYLD089) and CTR453. ( e ) Deconvoluted images of cultured ependymal cells stained with antibodies against CAP350 and TAP 952. ( f ) Deconvoluted images of cultured ependymal cells stained with antibodies against CYLD and TAP 952. Note that CYLD stained not only basal bodies but also cilia tips. Scale bars, 10 μm. Full size image To confirm the centrosomal localization of CYLD, we investigated its localization in multiciliated cells that contain numerous basal bodies. Serum starvation of cultured ependymal cells leads to the development of numerous motile cilia growing from these basal bodies [21] . Therefore, we cultured ependymal cells from mouse brains and stained them with antibodies against CAP350 and CYLD. Antibodies directed against glycylated tubulin, such as TAP952 (ref. 22 ) were used to decorate the cilia. Numerous dots located at the cilia base were labelled by antibodies directed against CAP350 or CYLD ( Fig. 2e,f ). A co-staining with antibodies directed against γ-tubulin suggests that both proteins localize at the basal bodies of multiciliated cells ( Supplementary Fig. 3 ). Surprisingly, CYLD antibodies, but not CAP350 antibody, stained the tips of the cilia and weakly the cilia themselves ( Fig. 2f ). Altogether, these results suggest that CYLD localizes at the centrosome and basal bodies but also at the ciliary tips. Truncated CYLD inhibits primary cilia formation The presence of CYLD at the basal bodies and at the ciliary tips prompted us to investigate the role of this protein in ciliogenesis. Therefore, we turned to Cyld Δ932 mice [23] , which express the smallest truncation of CYLD causing the human pathology (a deletion of the last 24 amino acids) leading to a catalytically inactive protein [24] ( Fig. 1a ). As previously described in mice with complete deletion of CYLD catalytic domain ( Cyld Δ9/Δ9 ) [19] , Cyld Δ932 mutants die perinatally from respiratory distress with pulmonary defects ( Supplementary Fig. 4 ) reminiscent of the phenotype observed in several mouse models exhibiting defects in signalling as Wnt5a [25] , Vangl2 (ref. 26 ) and GMAP210 (ref. 27 ). As these mutants show defects in cilia or in PCP signalling, we decided to investigate primary cilia formation in primary mouse embryonic fibroblasts (MEFs) derived from Cyld WT or Cyld Δ932 littermate embryos. We first verified that proliferation of cells of both genotypes was comparable as proliferation rate is likely to modify cell’s behaviour in respect to ciliation. Results of fluorescence-activated cell sorting (FACS) analysis or KI67 staining (a marker of proliferative cells) show that both WT and mutant MEFs proliferate similarly ( Supplementary Fig. 5a–c ). As CYLD is a tumour suppressor, and primary cilia usually form in the G0/G1 phase of the cell cycle [28] , we also wanted to determine whether both cell types were able to undergo cell cycle arrest on serum starvation. Again, after FACS analysis and KI67 staining we found no difference in the ratio of non-cycling cells between the two conditions ( Supplementary Fig. 5a–c ). Although both cell types proliferate similarly and are able to stop cycling on serum starvation, primary cilium staining showed that only 32% of Cyld Δ932 cells present a primary cilium compared with 68% of WT MEFs ( Fig. 3a,b ), suggesting that truncated CYLD mildly affects primary cilia formation. 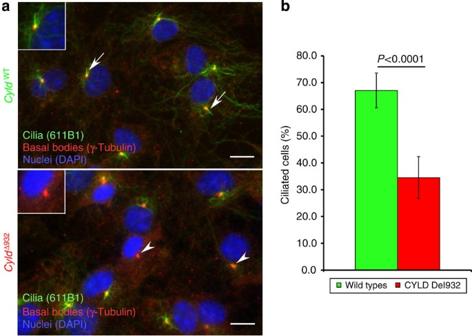Figure 3: CYLDΔ932affects primary cilia formation. (a) Staining of WT orCyldΔ932MEFs grown at confluence and serum depleted for 48 h with anti-acetylated tubulin (green) and anti-γ-tubulin (red) antibodies. WT MEFs cells show a primary cilium, while most of theCyldΔ932cells do not grow a primary cilium. Scale bars, 10 μm. (b) Quantification: a primary cilium was observed in about 68% of cells (n=ca.2,000 cells out of 4 embryos) of the WT MEFs, while only 32% of mutant cells (n=ca.4,000 cells out of 8 embryos) showed one.P-value <0.0001 afterχ2-test. Error bars show s.d. Figure 3: CYLD Δ932 affects primary cilia formation. ( a ) Staining of WT or Cyld Δ932 MEFs grown at confluence and serum depleted for 48 h with anti-acetylated tubulin (green) and anti-γ-tubulin (red) antibodies. WT MEFs cells show a primary cilium, while most of the Cyld Δ932 cells do not grow a primary cilium. Scale bars, 10 μm. ( b ) Quantification: a primary cilium was observed in about 68% of cells ( n = ca. 2,000 cells out of 4 embryos) of the WT MEFs, while only 32% of mutant cells ( n = ca. 4,000 cells out of 8 embryos) showed one. P -value <0.0001 after χ 2 -test. Error bars show s.d. Full size image Truncated CYLD inhibits multiple motile cilia formation We next examined motile cilia formation in trachea of WT and Cyld Δ932 E18.5 embryos from several litters by scanning electron microscopy. As ciliogenesis in the trachea occurs proximo-distally [29] , we imaged and counted the ciliated cells in every field from the larynx to the beginning of the main bronchi to avoid bias due to spatial differences. For each litter, the number of multiciliated cells was at least 50% lower in the mutants than in WT embryos. In addition, the motile cilia of mutant multiciliated cells were generally shorter and scarce ( Fig. 4a ). As a control of the specificity of this result, we took advantage of the previously published Cyld knock-out mouse model [18] , [30] , [31] . As Cyld KO mice live without any major health issues, we were not expecting any defects in cilia formation. Indeed, there was no difference in the morphology and number of multiciliated cells between the WT and Cyld KO embryos ( Fig. 4a , graph). These results show that CYLD Δ932 , a truncated catalytically inactive protein, behaves as a dominant negative form of CYLD to inhibit formation of motile cilia in multiciliated cells, whereas complete absence of CYLD has no effect on cilia formation. 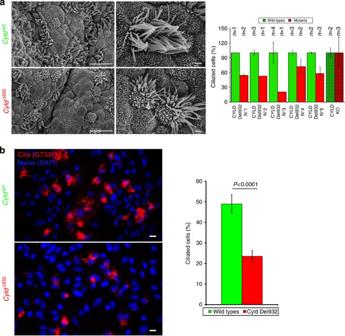Figure 4: CYLDΔ932affects multiple motile cilia formation. (a) Left: cilia analysis by scanning electron microscopy of tracheas isolated from WT andCyldΔ932embryos at E18.5. Representative fields of trachea from WT embryos (upper) orCyldΔ932mutant (lower) are shown, with a magnified image on the right. Right: quantification of the percentage of ciliated cells in the trachea from WT or mutant embryos. Analysis was performed on five litters fromCyldΔ932embryos and one litter fromCyldKOmice. The number of WT and mutant embryos is indicated at the top of each bar. The mean was determined when possible and the s.d. is indicated. Scale bars, 10 μm for the low magnification and 1 μm for the high magnification. (b) Left: staining of a large field of cultured ependymal cells isolated from WT (left) orCyldΔ932(right) from P0 animals 15 days after differentiation with GT335 for cilia and DAPI for nuclei. Note the decreased number of multiciliated cells in the mutant. Scale bars, 10 μm. Right: quantification of the percentage of multiciliated cells in WT orCyldΔ932cell cultures. Multiciliated cells in each culture were counted and reported relative to the number of nuclei. In mutant cell cultures, the number of multiciliated cells was reduced by 50%. (nfor WT=~2,500 cells of 5 embryos;nforCyldΔ932=~2,500 cells of 5 embryos).P-value <0.0001 afterχ2-test. Error bars show s.d. Figure 4: CYLD Δ932 affects multiple motile cilia formation. ( a ) Left: cilia analysis by scanning electron microscopy of tracheas isolated from WT and Cyld Δ932 embryos at E18.5. Representative fields of trachea from WT embryos (upper) or Cyld Δ932 mutant (lower) are shown, with a magnified image on the right. Right: quantification of the percentage of ciliated cells in the trachea from WT or mutant embryos. Analysis was performed on five litters from Cyld Δ932 embryos and one litter from Cyld KO mice. The number of WT and mutant embryos is indicated at the top of each bar. The mean was determined when possible and the s.d. is indicated. Scale bars, 10 μm for the low magnification and 1 μm for the high magnification. ( b ) Left: staining of a large field of cultured ependymal cells isolated from WT (left) or Cyld Δ932 (right) from P0 animals 15 days after differentiation with GT335 for cilia and DAPI for nuclei. Note the decreased number of multiciliated cells in the mutant. Scale bars, 10 μm. Right: quantification of the percentage of multiciliated cells in WT or Cyld Δ932 cell cultures. Multiciliated cells in each culture were counted and reported relative to the number of nuclei. In mutant cell cultures, the number of multiciliated cells was reduced by 50%. ( n for WT=~2,500 cells of 5 embryos; n for Cyld Δ932 =~2,500 cells of 5 embryos). P -value <0.0001 after χ 2 -test. Error bars show s.d. Full size image As the decreased number of multiciliated trachea cells might be due to a developmental delay in the Cyld Δ932 embryo, we used the ependymal culture system [21] and compared motile cilia formation in parallel cell cultures obtained from WT and Cyld Δ932 littermates. There was no difference in the doubling time of cells with these different genotypes, but there was a dramatic difference in the number of multiciliated cells between WT and Cyld Δ932 cells, independently of cell-density variations ( Fig. 4b ). Altogether, our results in trachea and ependymal cells culture show that truncation of the catalytic domain of CYLD affects formation of motile cilia of multiciliated cells. Cyld Δ932 basal bodies duplicate normally but fail to anchor To determine the reason of the decrease in cilia formation in Cyld Δ932 embryos, we studied basal body formation in ependymal cell cultures from each genotype at several differentiation time points by staining with antibodies specific for basal bodies and cilia. In WT cell cultures, multiciliated cells showed abundant basal bodies decorated with anti-centrin3 antibodies ( Fig. 5a ). Abundant basal bodies were also observed in Cyld Δ932 cells irrespective of the number of cilia in these cells. Quantification of cells with numerous basal bodies revealed only a slight decrease in Cyld Δ932 mutant cells, suggesting that basal bodies amplification proceeds similarly in WT and Cyld Δ932 cells ( Fig. 5a ). In addition, the timing of formation was not different between the two cell types. To further investigate a possible basal body defect, we performed detailed electron microscopy analysis of WT and mutant tracheas. We found that a significant number of basal bodies failed to position apically and dock at the plasma membrane in Cyld Δ932 tracheal ciliated cells ( Fig. 5b ). They appeared to be positioned in different orientation ( Fig. 5b , arrows). In addition, the microvilli, which interspaced the axonema, appeared to be reduced in length as well as in number, compared with the WT samples from the same litter, reminiscent of actin organization or Rho GTPase activity defect [32] , [33] . Thus, in mutant cells basal bodies multiply normally but fail to migrate apically, suggesting a defect in transport and/or docking at the apical membrane. 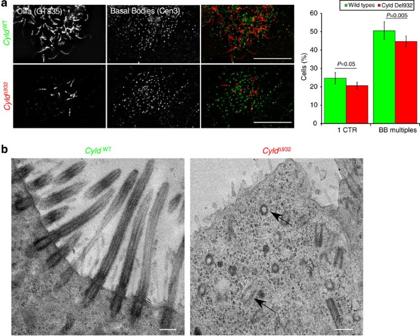Figure 5: CYLDΔ932affects basal body anchoring of motile cilia but not duplication. (a) Left: double-staining analysis of basal bodies and cilia in WT and mutant ependymal cell cultures using GT335 and antibodies against Centrin 3, 15 days after serum removal. WT orCyldΔ932multiciliated cells show a large number of basal bodies irrespective of the presence or absence of cilia. Images have been deconvoluted. Scale bars, 10 μm. Right: quantification of the number of cells with multiple basal bodies and cells with a centrosome in WT and mutant ependymal cell cultures. Mutant cells showed a slight but significant decrease in the number of cells with multiple basal bodies compared with the WT culture. A slight decrease was also observed in the number of cells showing a centrosome. (~1,900 cells of four WT embryos; ~1,900 cells of fourCyldΔ932embryos.)P-values afterχ2-test are <0.05 and 0.005, respectively. Error bars show s.d. (b) Transmission electron microscopy image of WT (left) orCyldΔ932(right) trachea. In the WT trachea, numerous regularly spaced anchored basal bodies are evident at the apical membrane. All of them show an axoneme. In the mutant trachea, duplicated basal bodies are organized in several orientations; some are transversally oriented, while others are longitudinally oriented (arrows). In addition, although some microvilli are observed on the apical surface most of the cells do not show any microvilli at their surface. Scale bars, 500 μm. Figure 5: CYLD Δ932 affects basal body anchoring of motile cilia but not duplication. ( a ) Left: double-staining analysis of basal bodies and cilia in WT and mutant ependymal cell cultures using GT335 and antibodies against Centrin 3, 15 days after serum removal. WT or Cyld Δ932 multiciliated cells show a large number of basal bodies irrespective of the presence or absence of cilia. Images have been deconvoluted. Scale bars, 10 μm. Right: quantification of the number of cells with multiple basal bodies and cells with a centrosome in WT and mutant ependymal cell cultures. Mutant cells showed a slight but significant decrease in the number of cells with multiple basal bodies compared with the WT culture. A slight decrease was also observed in the number of cells showing a centrosome. (~1,900 cells of four WT embryos; ~1,900 cells of four Cyld Δ932 embryos.) P- values after χ 2 -test are <0.05 and 0.005, respectively. Error bars show s.d. ( b ) Transmission electron microscopy image of WT (left) or Cyld Δ932 (right) trachea. In the WT trachea, numerous regularly spaced anchored basal bodies are evident at the apical membrane. All of them show an axoneme. In the mutant trachea, duplicated basal bodies are organized in several orientations; some are transversally oriented, while others are longitudinally oriented (arrows). In addition, although some microvilli are observed on the apical surface most of the cells do not show any microvilli at their surface. Scale bars, 500 μm. Full size image Centriole maturation and satellites are not affected The failure of basal bodies to anchor could be explained by either a defect in centriole maturation or in centriolar satellite organization. Indeed, centriolar maturation is characterized by the acquisition of subdistal and distal appendages, which form the ciliary basal feet and transition fibres, respectively [34] . Both of them are required for cilia formation. Furthermore, centriolar satellites are believed to drive cargo to the centrosome and basal bodies [35] , and are also required for ciliogenesis [36] . To ascertain the presence of centriolar satellites and appendages, we stained ependymal cells with antibodies directed against PCM1 and OFD1, two proteins of centriolar satellites [35] , [36] , as well as with antibodies against Cep164 and CCDC123 (Cep123), two proteins located within the distal appendages [37] , [38] , and ODF2, a protein located both at distal and subdistal appendages [39] . All antibodies decorated centriolar satellites or basal bodies irrespective of the genotype ( Fig. 6 ), suggesting that basal body maturation and centriolar satellite organization are not significantly modified in Cyld Δ932 mice. 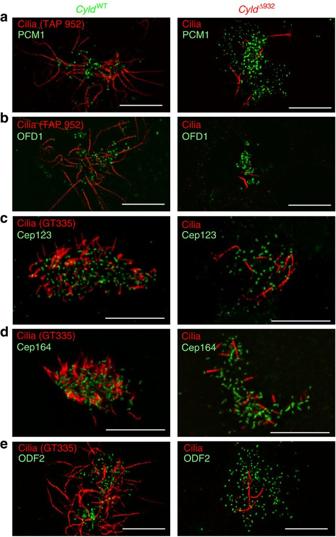Figure 6: Centriolar satellite organisation and centriole maturation is not affected inCyldΔ932ependymal cells. Staining for cilia (TAP 952), the centriolar satellite protein PCM1 (a) and OFD1 (b) in WT (left) orCyldΔ932(right) ependymal cells. Staining for cilia (GT335) and the centriole appendages proteins Ccdc123 (Cep123) (c), Cep164 (d) and ODF2 (e). Cilia are in red and PCM1, OFD1, Cep123, Cep164 and ODF2 are in green. Scale bars, 10 μm. Figure 6: Centriolar satellite organisation and centriole maturation is not affected in Cyld Δ932 ependymal cells. Staining for cilia (TAP 952), the centriolar satellite protein PCM1 ( a ) and OFD1 ( b ) in WT (left) or Cyld Δ932 (right) ependymal cells. Staining for cilia (GT335) and the centriole appendages proteins Ccdc123 (Cep123) ( c ), Cep164 ( d ) and ODF2 ( e ). Cilia are in red and PCM1, OFD1, Cep123, Cep164 and ODF2 are in green. Scale bars, 10 μm. Full size image Cyld Δ932 does not interact with CAP350 To gain molecular insight into the defects associated with CYLD Δ932 expression, we tested whether CYLD Δ932 protein interacted with CAP350 by immunoprecipitation of CAP350 in WT and Cyld Δ932 MEFs. In parallel experiments, CAP350 antibody immunoprecipitated CYLD (revealed by a polyclonal antibody directed against the amino-terminal domain) in WT but not Cyld Δ932 MEFs ( Fig. 7 ), suggesting that the truncated version of CYLD is unable to interact with CAP350. It follows that CYLD Δ932 would not be localized at the centrosome and, indeed, we did not detect any CYLD at the centrosome or basal bodies in Cyld Δ932 mutant ependymal cells ( Fig. 7b,c ), while CAP350 remained at the centrosome. It is worth noting that CYLD was still localized at the ciliary tip in mutant ependymal cells. These observations indicate that the lack of interaction between CYLD Δ932 and CAP350 results in abnormal CYLD localization. 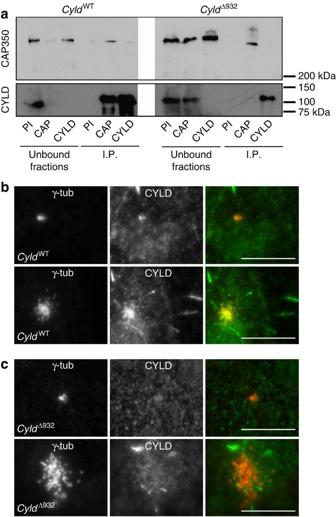Figure 7: CYLDΔ932does not interact with CAP350 and does not localize at the centrosome. (a) Immunoprecipitation of WT orCyldΔ932MEFs cells using rabbit pre-immune (PI), anti-CAP350 (polyclonal) and CYLD 089 (polyclonal) IgG. The immunoprecipitated proteins and non-associated components are labelled ‘Immunoprecipitate (I.P.)’ and ‘Unbound fraction’, respectively. I.P. results were analysed by WB analysis using antibodies against CAP350 and CYLD (polyclonal). In WT cells, CAP350 immunoprecipitated CYLD (revealed by the polyclonal antibody (089) confirming the results obtained onFig. 1a). However, we did not observe any CYLD in the CAP350 immunoprecipitates ofCyldΔ932MEFs. CAP, CAP350. (b,c) CYLD localization in WT (b) orCyldΔ932(c) MEFs (upper panel) or ependymal cells (lower pannel). CYLD localizes at the centrosome and basal bodies in WT cells, while CYLDΔ932no longer localizes at the centrosome or basal bodies. Scale bars, 10 μm. Figure 7: CYLD Δ932 does not interact with CAP350 and does not localize at the centrosome. ( a ) Immunoprecipitation of WT or Cyld Δ932 MEFs cells using rabbit pre-immune (PI), anti-CAP350 (polyclonal) and CYLD 089 (polyclonal) IgG. The immunoprecipitated proteins and non-associated components are labelled ‘Immunoprecipitate (I.P. )’ and ‘Unbound fraction’, respectively. I.P. results were analysed by WB analysis using antibodies against CAP350 and CYLD (polyclonal). In WT cells, CAP350 immunoprecipitated CYLD (revealed by the polyclonal antibody (089) confirming the results obtained on Fig. 1a ). However, we did not observe any CYLD in the CAP350 immunoprecipitates of Cyld Δ932 MEFs. CAP, CAP350. ( b , c ) CYLD localization in WT ( b ) or Cyld Δ932 ( c ) MEFs (upper panel) or ependymal cells (lower pannel). CYLD localizes at the centrosome and basal bodies in WT cells, while CYLD Δ932 no longer localizes at the centrosome or basal bodies. Scale bars, 10 μm. Full size image CYLD localization and activity are required for ciliogenesis As the impaired ciliogenesis observed in Cyld Δ932 mice might be driven by the absence of CYLD at the centrosome, or by its compromised catalytic activity or both, we decided to investigate the effect of CYLD activity and localization on primary cilia formation. This was performed by overexpressing CYLD WT as well as its catalytically inactive version CYLD H871/N (ref. 24 ) in RPE1 cells. Overexpressed CYLD WT or CYLD H871/N protein is mainly cytosolic with no obvious enrichment at the centrosome ( Fig. 8a ). We observed a dramatic decrease in primary cilia formation in cells expressing GFP-CYLD WT , CYLD WT -Flag or CYLD H871/N -Flag ( Fig. 8a ) with 23%, 17% and 24% of ciliated cells, respectively, while non-transfected cells or green fluorescent protein (GFP)-transfected cells showed ~90%. 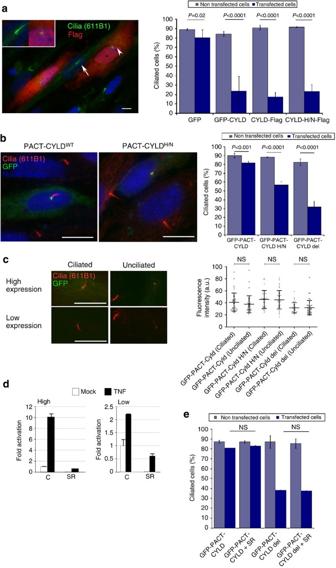Figure 8: Regulation of primary cilium formation by CYLD in an NF-κB-independent manner. (a) Left, immunostaining of cells overexpressing CYLD-Flag; red, anti-Flag antibodies; green, anti-acetylated tubulin antibodies. Non-transfected cells show a primary cilium (arrow), while cells transfected with CYLD-Flag show only the centrosome (arrowhead). Scale bars, 10 μm. Right: percentage of ciliated cells. Untransfected and GFP-transfected cells show a similar percentage of ciliated cells. Fewer cells are ciliated after transfection with GFP-CYLD, CYLD-Flag or CYLD H/N-Flag. For each condition, at least 500 cells in 3 experiments were counted.P-values afterχ2-test are 0.02 for GFP and <0.0001 for the three other conditions. (b) Left: immunostaining of cells overexpressing GFP-PACT-CYLDWTor GFP-PACT-CYLDH/N. Red, anti-acetylated tubulin antibodies; green, GFP. Scale bars, 10 μm. Right: percentage of ciliated cells expressing GFP-PACT-CYLDWT, GFP-PACT-CYLDH/Nand GFP-PACT-CYLDΔ932. The targeting of CYLDWTto the centrosome does not affect ciliogenesis unless the catalytic domain is not functionnal (GFP-PACT-CYLDH/Nand GFP-PACT-CYLDΔ932). For each condition, at least 500 cells in 3 experiments were counted.P-values afterχ2-test are <0.001 for GFP-PACT-CYLD and <0.0001 for the other conditions. (c) Left: cells with high expression level or low expression level of the H/N construct can be ciliated or unciliated. Cells were transfected with GFP-PACT-CYLD H/N (green) and stained with anti-acetylated tubulin antibody (red). Right: average fluorescence intensity (arbitrary units) measured at the centrosome for ciliated and unciliated cells after transfection of the three constructs (GFP-PACT-CYLDWT, GFP-PACT-CYLDH/Nor GFP-PACT-CYLDΔ932=GFP-PACT-Cyld del) in RPE1 cells. Mean and s.d. are shown. Differences after Mann–Whitney’s test are not statistically significant (n.s;P=0.3;P=0.9 andP=0.65, respectively). (d) Ig-κB-Luciferase-derived activity measured after culture of cells in high or low serum medium. In each case both basal (Mock) and induced (TNF) levels of NF-κB activity were strongly inhibited by IκBα-SR. Errors bars in all graphs show s.d. (e) Percentage of ciliated cells in GFP-PACT-CYLDWT, GFP-PACT-CYLDH/Nand GFP-PACT-CYLDΔ932after inhibition of the NF-κB signalling by expression or not of the Super-repressor IκBα. It is worth noting that afterχ2-test statistically significant differences can be observed irrespective of the PACT-CYLD fusion construct after NF-κB inhibition. Figure 8: Regulation of primary cilium formation by CYLD in an NF-κB-independent manner. ( a ) Left, immunostaining of cells overexpressing CYLD-Flag; red, anti-Flag antibodies; green, anti-acetylated tubulin antibodies. Non-transfected cells show a primary cilium (arrow), while cells transfected with CYLD-Flag show only the centrosome (arrowhead). Scale bars, 10 μm. Right: percentage of ciliated cells. Untransfected and GFP-transfected cells show a similar percentage of ciliated cells. Fewer cells are ciliated after transfection with GFP-CYLD, CYLD-Flag or CYLD H/N-Flag. For each condition, at least 500 cells in 3 experiments were counted. P -values after χ 2 -test are 0.02 for GFP and <0.0001 for the three other conditions. ( b ) Left: immunostaining of cells overexpressing GFP-PACT-CYLD WT or GFP-PACT-CYLD H/N . Red, anti-acetylated tubulin antibodies; green, GFP. Scale bars, 10 μm. Right: percentage of ciliated cells expressing GFP-PACT-CYLD WT , GFP-PACT-CYLD H/N and GFP-PACT-CYLD Δ932 . The targeting of CYLD WT to the centrosome does not affect ciliogenesis unless the catalytic domain is not functionnal (GFP-PACT-CYLD H/N and GFP-PACT-CYLD Δ932 ). For each condition, at least 500 cells in 3 experiments were counted. P -values after χ 2 -test are <0.001 for GFP-PACT-CYLD and <0.0001 for the other conditions. ( c ) Left: cells with high expression level or low expression level of the H/N construct can be ciliated or unciliated. Cells were transfected with GFP-PACT-CYLD H/N (green) and stained with anti-acetylated tubulin antibody (red). Right: average fluorescence intensity (arbitrary units) measured at the centrosome for ciliated and unciliated cells after transfection of the three constructs (GFP-PACT-CYLD WT , GFP-PACT-CYLD H/N or GFP-PACT-CYLD Δ932 =GFP-PACT-Cyld del) in RPE1 cells. Mean and s.d. are shown. Differences after Mann–Whitney’s test are not statistically significant (n.s; P =0.3; P =0.9 and P =0.65, respectively). ( d ) Ig-κB-Luciferase-derived activity measured after culture of cells in high or low serum medium. In each case both basal (Mock) and induced (TNF) levels of NF-κB activity were strongly inhibited by IκBα-SR. Errors bars in all graphs show s.d. ( e ) Percentage of ciliated cells in GFP-PACT-CYLD WT , GFP-PACT-CYLD H/N and GFP-PACT-CYLD Δ932 after inhibition of the NF-κB signalling by expression or not of the Super-repressor IκBα. It is worth noting that after χ 2 -test statistically significant differences can be observed irrespective of the PACT-CYLD fusion construct after NF-κB inhibition. Full size image As this result could be due to aberrant CYLD localization, we decided to force CYLD expression at the centrosome using the centrosomal targeting domain, PACT [40] . The targeting of this GFP-PACT-CYLD WT to the centrioles affected ciliogenesis only slightly, resulting in ~80% of ciliated cells ( Fig. 8b ). By contrast, the targeting to the centrioles of CYLD with a point mutation, which impaired the catalytic activity of CYLD (GFP-PACT-CYLD H871/N ), showed only 57% of ciliated cells. A similar decrease was also observed ( Fig. 8b , graph) when using the truncated and catalytically inactive version of CYLD, GFP-PACT-CYLD Δ932 (ref. 24 ). To control that these observations are not caused by differences in the expression level of the constructs, we measured GFP fluorescence intensity at the centrosome for each condition in a new experiment. General observation of the slides showed similar differences in cell ciliation of transfected cells (ciliated cells: GFP-PACT-CYLD WT (82%), GFP-PACT-CYLD H871/N (60%), GFP-PACT-CYLD Δ932 (36%)), but no significant difference in mean fluorescence intensity was observed between ciliated and unciliated cells, irrespective of the construct, which shows that ciliation is independent of expression level ( Fig. 8c ). These results demonstrate that both the localization of CYLD at the centrosome/basal body and its deubiquitinase activity are essential for its function in ciliogenesis. Ciliogenesis defects are independent of NF-κB activation As CYLD is a negative regulator of the NF-κB signalling pathway, we were wondering whether the defective ciliogenesis observed on the trachea and ependymal cells of mutant mice or after targeting at the centrosome catalytically inactive CYLD, might be due to a deregulation of the NF-κB pathway. Therefore, we decided to co-transfect RPE1 cells with either GFP-PACT-CYLD WT or GFP-PACT-CYLD Δ932 with or without a non-degradable form of IκB acting a Super-repressor of NF-κB (IκBα Super-Repressor (IκBα-SR)) [41] to block NF-κB activation. As shown on Fig. 8d , the addition of the tumour necrosis factor (TNF) induced activation of NF-κB either in the presence of serum or after 48 h serum depletion, while the presence of IκBα-SR completely blocked this activation. In parallel, cells were fixed and analysed for the presence of a primary cilium. Expression of IκBα-SR did not impact the ciliation process either in GFP-PACT-CYLD WT - or in GFP-PACT- CYLD Δ932 -expressing cells as shown in Fig. 8e , suggesting that the defects in the ciliogenesis process due to the presence of GFP-PACT-CYLD Δ932 at the centrosome is independent of NF-κB signalling. In this study we demonstrate that part of the CYLD pool is located at the centrosome/basal bodies, through its interaction with CAP350. This interaction is attested by several observations. First of all, we identified CYLD by mass spectrometry as a partner of CAP350 and confirmed their interaction in endogenous immunoprecipitation experiments; Furthermore, we demonstrate by co-overexpression that the C-terminal portion of CYLD, including the DUB domain, interacts with the C-terminal domain of CAP350. Second, CAP350 overexpression directs the centrosomal localization of overexpressed CYLD; finally, CYLD no longer localizes at the centrosome when its interaction with CAP350 is abolished. It is worth noting that CYLD has already been found in interaction with another centrosomal protein CEP192 in co-overexpressed conditions, reinforcing the centrosomal localisation of CYLD [16] . Nevertheless, the relationship between CAP350/CEP192 and CYLD will require further investigations. This specific centrosomal localization combined with the staining observed at the tip of motile cilia suggests that CYLD plays a role in cilia assembly/disassembly. Interestingly, localization of CYLD at the cilia tips is reminiscent of the enrichment observed for several other proteins such as EB1/EB3 (ref. 42 ), some IFT proteins [43] and, more recently, cep104/FAP256 (ref. 44 ). This localization of CYLD is probably independent of its DUB activity, as the staining at the cilia tip is still observed in Cyld Δ932 ependymal cells. As a matter of fact, an interaction between CYLD and EB1 has recently been reported [45] . In any case, this dual CYLD localization at the centrosome and at the cilia tip suggests that CYLD has distinct functions depending on the partners it interacts with. Our results show that CYLD participates in ciliogenesis by allowing basal bodies to migrate and dock to the plasma membrane. However, not all motile cilia are affected, as CYLD Δ932 mutants do not display any left–right patterning defects, suggesting that the function of the node is unaffected by CYLD truncation. In addition, we demonstrate that CYLD has to be both catalytically active and located at the centrosome to promote ciliogenesis. Therefore, we propose a model ( Fig. 9 ) in which ciliogenesis would be only possible if a centrosomal protein, or CAP350 itself, is deubiquitinated. In the WT situation, CYLD would be located at the centrosome/basal body via CAP350 and be able to hydrolyse K63- or linear-linked ubiquitin chains from its substrate, enabling ciliogenesis to proceed. In the mutant situation, CYLD would not be present at the centrosome, resulting in impaired ciliogenesis. On CYLD overexpression, extra CYLD in the cytoplasm would delocalize its targets and prevent ciliogenesis. However, when CYLD is overexpressed and targeted to the basal body by the PACT domain, it can deubiquitinate its target and, consequently, ciliogenesis occurs. Conversely, cells overexpressing the catalytically inactive CYLD H871/N or CYLD Δ932 fused with the PACT domain do not retain the ability to develop cilia. All these results argue for the involvement of K63-ubiquitination/deubiquitination in ciliogenesis. Importantly, we demonstrate that this role is NF-κB independent. Recently, several reports have suggested an inhibition of ciliogenesis caused by activation of the NF-κB pathway. First, Lattke et al. [46] have shown that the activation of this pathway by the expression of constitutively active IKK2 inhibits cilia formation. However, it is not clear whether the cilia formation defect is a consequence of a direct cell-autonomous NF-κB activation rather than activation of inflammatory processes. Moreover, it could also be a direct effect of active IKK2 in ependymal cells, independently of NF-κB, as IKK2 has NF-κB-independent functions [47] . As a matter of fact, IKK2 has been found inhibiting ciliogenesis in an RNA interference screen [48] . Second, the pro-inflammatory cytokine TNF triggered a dose-dependent loss of primary cilia in mesenchymal stromal cells [49] , but no molecular explanation was provided. However, our study brings several arguments supporting the fact that this DUB acts on ciliogenesis independently of NF-κB activation as trachea from CYLD KO mice do not show any defects in motile cilia formation, whereas they are defective in NF-κB signalling [14] , [18] , and inhibition of the NF-κB pathway by the expression of a non-degradable form of IκBα acting as a Super-repressor [41] do not modify the ciliogenesis defect caused by expression of the CYLD Δ932 protein at the centrosome. 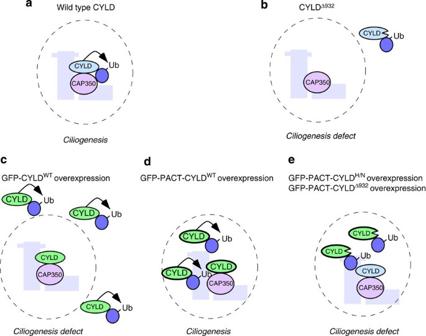Figure 9: Model explaining CYLD function at the centrosome. (a) In WT mice, CYLD is located at the centrosome and can deubiquitinate its target to promote ciliogenesis. (b) In mutant mice (CyldΔ932), CYLD is no longer located at the centrosome and cannot deubiquitinate its target preventing ciliogenesis. (c) After CYLD overexpression, extra CYLD is found in the cytoplasm and will delocalize its target from the centrosome. A ciliogenesis defect is observed. (d) Targeting of CYLD to the centrosome by the PACT domain (GFP-PACT-CYLD), allow CYLD to deubiquitinate its targets and ciliogenesis to occur. (e) In contrast, targeting of catalytically inactive CYLD to the centrosome by the PACT domain (GFP-PACT-CYLDH/Nor GFP-PACT-CYLDΔ932) prevents ciliogenesis. In these cases, targets cannot be deubiquitinated and ciliogenesis defects are observed. Overexpressed CYLD is displayed in green, CYLD fused to the PACT domain is encircled with a bolder line. Figure 9: Model explaining CYLD function at the centrosome. ( a ) In WT mice, CYLD is located at the centrosome and can deubiquitinate its target to promote ciliogenesis. ( b ) In mutant mice ( Cyld Δ932 ), CYLD is no longer located at the centrosome and cannot deubiquitinate its target preventing ciliogenesis. ( c ) After CYLD overexpression, extra CYLD is found in the cytoplasm and will delocalize its target from the centrosome. A ciliogenesis defect is observed. ( d ) Targeting of CYLD to the centrosome by the PACT domain (GFP-PACT-CYLD), allow CYLD to deubiquitinate its targets and ciliogenesis to occur. ( e ) In contrast, targeting of catalytically inactive CYLD to the centrosome by the PACT domain (GFP-PACT-CYLD H/N or GFP-PACT-CYLD Δ932 ) prevents ciliogenesis. In these cases, targets cannot be deubiquitinated and ciliogenesis defects are observed. Overexpressed CYLD is displayed in green, CYLD fused to the PACT domain is encircled with a bolder line. Full size image Nevertheless, it is intriguing that Cyld KO mice are perfectly viable without any problem in motile cilia formation, whereas the mice expressing a truncated version of CYLD die at birth with cilia defects. These results suggest some redundancy in the control of ciliogenesis by DUBs. In the Cyld KO mice another DUB may compensate for the function of CYLD, whereas in the Cyld Δ932 mice the mutant CYLD protein probably acts as a dominant negative by delocalizing its substrate, thus preventing the action of the substitute DUB. USP 21 is a good candidate for carrying this function, as it has recently been shown to localize at the centrosome and affect primary cilia formation [50] . Moreover, it shares a similar target with CYLD in the regulation NF-κB signalling pathway [51] . The involvement of the deubiquitinase CYLD in basal body migration/docking has to be integrated in a more general role of ubiquitination processes in ciliogenesis or centrosomal function. At first, ubiquitinated proteins have been reported to be present in cilia and flagella [52] , and the K63-specific E2 ubiquitin-conjugating enzyme Ubc13 is present in the ciliome of various species [52] , [53] , [54] , [55] . Next, protein ubiquitination was involved in flagellar disassembly [52] . Finally, the E3 ubiquitin ligase MIB1 (ref. 56 ) was identified in a centrosome proteome [57] and the deubiquitinase USP21 is shown to be required for primary cilia formation [50] . In addition, another deubiquitinase Usp33 has recently been shown to localize at the centrosome by its binding with CP110 and its activity antagonizes SCF cyclinF ubiquitination of CP110 (ref. 58 ). How may CYLD regulate ciliogenesis? Our data show that CYLD is required to allow basal body migration and docking at the plasma membrane. We also show that centriole maturation proteins as well as some centriolar satellite proteins are still present in our mutants, suggesting that the anchoring defect is not a result of basal body structural defects. However, we cannot rule out that ubiquitination/deubiquitination processes might affect centriole appendages and centriolar satellite functions [59] , [60] . Interestingly, a target of CYLD, Dvl [15] , has been shown in Xenopus multiciliated cells to be essential for the positioning of the apical basal bodies and for the activation of the Rho GTPase [61] . In addition, the RhoGEF LARG, co-immunoprecipitates with CYLD [62] . Therefore, we propose that CYLD would allow basal body migration by deubiquitinating, a substrate working with Dvl, and LARG to activate RhoA GTPase and subsequently remodel actin. The recent report that phosphorylated CYLD redistributes to the dorsal ruffles [63] supports this hypothesis of a link between CYLD and the actin network. In conclusion, our work identifies CYLD as a new regulator of ciliogenesis. Two recent studies [64] , [65] have recently reported that impaired ciliogenesis impacts skin homeostasis and affects the pilosebaceous unit from which cylindroma are believed to originate. This convinced us that future studies designed to precisely characterize the molecular pathways regulated by CYLD during ciliogenesis might provide novel insights into how CYLD deregulation results in cylindroma in the cylindromatosis pathology. Mice All animals were housed in specific pathogen-free conditions at Institut Curie according to French and European Union laws. All animal procedures were conducted in accordance with European, national and institutional guidelines and protocols, and were approved by local government authorities (Authorization for animal testing N°91-518, Direction départementale des services vétérinaires de l’Essonne). Cyld Δ932 and Cyld KO mice were generated in a c57/Bl6J background as described previously [23] , [30] . Male and female embryos were used. As no differences between Cyld Δ932 heterozygous mice or embryos and their WT littermates were observed throughout the study, we pooled the results of both genotypes under the classification of WT. The embryonic stage was estimated on the basis of gestational time, with day 0.5 being defined as the morning when a vaginal plug was detected. Adult mice and embryos were genotyped by PCR. Cell culture Human retinal pigment epithelial (RPE1) cells were obtained from ATCC and grown in DMEM/F12 medium supplemented with 10% FCS. Human lymphoblastic KE37 cells obtained from M. Bornens’s laboratory were grown in RPMI medium supplemented with 10% FCS. MEFs were obtained after trypsinization of dissected embryos at embryonic day 13.5 (E13.5) and grown in DMEM medium supplemented with 10% FCS and non-essential amino acids. Ependymal cell cultures were maintained as described previously [21] , [66] . Human embryonic kidney cells (HEK293T) from ThermoScientific were transiently transfected with plasmid DNA using the calcium phosphate precipitation method. RPE1 cells were transiently transfected with plasmid DNA using X-tremeGENE HP (Roche) or Nucleofection (Amaxa) and fixed 24–48 h after transfection. Cellular fractionation Centrosomes were isolated from KE37 cells as described previously [67] . Briefly, cells were pretreated for 1 h with Nocodazole (2 × 10 −7 M) and Cytochalasin D (1 μg ml −1 ). Cells were washed in PBS and resuspended in 8% sucrose in ten times diluted PBS before cell lysis in lysis buffer (1 mM HEPES, 0.5 mM MgCl 2 , 0.5%NP40, 1 mM phenylmethanesulphonyl fluoride and anti-proteases). After centrifugation at 2,500 g , the supernatant is filtered through a nylon-mesh and readjusted to 10 mM HEPES and treated with DNAse. Concentrated centrosomes were overlaid on a discontinuous sucrose gradient (70%, 50% and 40%) in a SW28 tube and centrifuged for 1 h 15 min at 26,000 r.p.m. Fractions were collected and analysed for centrosomes. One percent Triton X-100 soluble or insoluble cell fractions were isolated from KE37 or RPE1 cells as described by Tassin et al. [68] Plasmid construction Full-length CAP350 and CYLD cDNAs were subcloned into a GFP vector (GFP-C3 from Clontech) for expression of GFP-tagged proteins. Different fragments of CAP350 cDNAmyc-tagged corresponding to AA 1-893, 984-2589 and 2590-3117 were previously described [8] . The CYLD-Flag construct was previously described [24] . The ΔC CYLD construct was designed by introducing a stop codon in AA 586. The PACT domain was amplified from human AKAP450 and then subcloned into the GFP-CYLD vectors. All constructions have been verified by sequencing. Antibodies Three antibodies directed against CYLD were used: a polyclonal antibody obtained by immunizing rabbits against the N-terminal region (amino acids 1–555) of CYLD (CYLD 089) and affinity purified (diluted 1/1,000 for WB analysis and 1/300 for immunofluorescence (IF), a monoclonal antibody directed against the full-length CYLD supplied by Millipore, which does not recognize endogenous protein from RPE1 and HEK293T cells (diluted 1/500 for WB analysis) and a monoclonal antibody supplied by Santa Cruz Biotechnology (E-10, SC-74435) recognizing the catalytic domain of the protein (diluted 1/100 for WB analysis). All antibodies have been characterized by the following procedure: they are recognized by WB analysis and IF overexpressed GFP-CYLD, as well as the immunoprecipitated protein. However, the polyclonal one gave a stronger signal both in IF and WB analysis. Two antibodies directed against γ-tubulin were used: a previously described polyclonal antibody [68] (1/500) and a monoclonal one (GTU88 from Sigma 1/1,000). We also used affinity-purified rabbit polyclonal antibodies directed against Centrin 3 (ref. 69 ) (1/1,000), CAP350 (ref. 8 ) (1/1,000), Ccdc123 (ref. 38 ) (1/250), Cep 164 (ref. 37 ) (1/1,000), PCM1 (ref. 70 ) (1/1,000), OFD1 (residues 145–1,012) [36] (1/100), ODF2 (residus 250–632) [48] (1/1,000) and several anti-tubulin antibodies were used, such as detyrosinated tubulin (T12)(1/1,000), polyglutamylated-tubulin (GT335) (1/50,000) and monoglycylated tubulin (TAP) (1/50,000) as described in Janke and Bulinski [22] . Antibodies against acetylated tubulin (clone 6-11 B 1) (1/1,000) and tubulin (clone B5-1-2) were purchased from Sigma and rabbit anti-Ki67 (1/500) (Novocastra Laboratories). DAPI (4′,6-diamidino-2-phenylindole, Sigma) was used for DNA labelling. In all experiments using Flag antibodies, we used the anti-flag M2 from Sigma (F1804)(1/1,000). Only the WB analysis of the ΔN CYLD was revealed by Rabbit anti-Flag antibodies (F7425) (1/500). Western blotting Protein extracts were run on a PAGE gel of various acrylamide/bisacrilamyde percentages. Gels were transferred on nitrocellulose membranes with a semi-dry transfer device (Bio-Rad). Membranes were then blotted with various antibodies then revealed by electrochemiluminescence on autoradiographs. Non-cropped scans of the autoradiograps of the main WB analysis are presented in Supplementary Fig. 6 . IF microscopy and data processing Cells were either fixed with methanol for 6 min at −20 °C and permeabilized for 30 s in PHEM buffer containing 0.25% Triton X-100 before methanol fixation or fixed with 4% paraformaldehyde for 15 min before permeabilization with 1% Triton X-100 and processed for IF as described previously [68] . After immunostaining, three-dimensional microscopy was performed using an upright motorized microscope (DM RXA2, Leica Microsystems, Mannheim, Germany) equipped with an oil immersion × 40, × 63, × 100/numerical aperture 1.4 Plan-Apochromat objective lens and a cooled interline charge-coupled device detector (Photometrics Coolsnap HQ). Z -positioning was accomplished using a piezoelectric driver (LVPZT, Physik Instruments, Waldbronn, Germany) mounted underneath the objective lens. The whole system operated using Metamorph software (Universal Imaging Corp., Downingtown, PA). Z -stacks were generated from optical sections taken at 0.2-μm intervals. Z -stacks were deconvoluted using Metamorph software with the appropriate point spread function (PSF) and Meinel algorithm. In Fig. 8c , pictures were taken with a wide-field fluorescence microscope (Zeiss Axiovert 200 M equipped with an Hamammatsu C4742 camera). For each picture in the GFP channel, all parameters were kept identical (exposure time, binning, camera gain, Offset and so on). Average pixel fluorescence intensity of GFP at the centrosome was then measured within a defined and constant circular area of the size of a centriole, using the measurement tools of Image J. Quantification data were compiled from measurements of 80 cells from each of the 3 constructs. Raw measurements for each 80 cells are plotted along the y axis in the graph to make comparison easier. Immunoprecipitation experiments Proteins from RPE1, HEK293T or MEF cells were extracted with 1D buffer [15] , [68] . After a centrifugation to eliminate trace aggregates, primary antibodies preadsorbed to protein G-sepharose beads (Pharmacia) were added to the sample and the mixture incubated for 2 h at 4 °C. Protein G-sepharose beads were then sedimented. The sedimented protein G-sepharose beads were washed (five times) with buffer and supernatants were precipitated with cold methanol. Proteins were then processed for SDS–PAGE electrophoresis and WB analysis. For mass spectrometry analysis, the protein spots were excised from the gel after coloration with colloidal Coomassie blue (G250; Bio-Rad), reduced using dithiothreitol and alkylated using iodoacetamide. The proteins were subjected to digestion with trypsin (Sigma). The extracted peptides were analysed by matrix-assisted laser desorption-ionization–time of flight mass spectrometry (Voyager-DETM PRO, Applied Biosystems). Peptide masses obtained by this analysis were used to search the National Center for Biotechnology Information database to identify the full-length proteins. Scanning electron microscopy Tracheas were dissected from embryos at embryonic day 18.5 (E18.5), fixed overnight in 2.5% glutaraldehyde/2% paraformaldehyde in 0.1 M sodium cacodylate buffer pH 7.2 and post-fixed with 2% osmium tetroxide (Electron Microscopy Sciences). Samples were dehydrated in a graded ethanol series and dried with hexamethyldisilazane (HMDS) or the CO 2 critical point dryer Leica CPD-030. Specimens were coated with 10 nm gold/palladium in a Gatan Ion Beam Coater 681 and observed in a field emission scanning electron microscope JSM-6700f (JEOL, Japan). Image processing and analyses were performed with ImageJ software. Transmission electron microscopy Tracheas were dissected from embryos at E18.5, fixed overnight in 2.5% glutaraldehyde/2% paraformaldehyde in 0.1 M sodium cacodylate buffer pH 7.2 and post-fixed with 2% osmium tetroxide. Samples were dehydrated in a graded ethanol series and embedded in Epon (Electron Microscopy Science). Longitudinal 200-nm-thick sections were prepared with an ultramicrotome (Leica) and mounted on copper grids (200 mesh). The samples were observed in a 200-kV field emission gun electron microscope with an in-column energy filter (omega filter) JEM 2200 FS (JEOL, Japan). Cilia counting and statistics As ciliated cells in the trachea differentiate proximo-distally, we counted the cells in a series of jointed pictures taken from the larynx to the main bronchi to avoid any bias based on differentiation time. For a better visualization, results were normalized. This was achieved by taking the number of ciliated cells of WT embryos as 100%. In MEF cell cultures, primary cilia formation is not always homogeneous. Therefore, we took the pictures for counting in a randomized manner, observing the centrosome. The same field was then examined for the presence of cilia. Most of the experiments needing statistical validation involved paired observations on two variables for which we wanted to assess the independence of two populations. In those cases, the events being considered were mutually exclusive and the total probability was one. All observations were independent. Therefore, we used Fisher’s exact test or, when the sample sizes were large enough to avoid a type II error following Cochran’s rules, we performed Pearson’s χ 2 -test without Yates’ correction. All calculations were made with GraphPad Prism 5. Statistical significance in the fluorescence intensity experiment ( Fig. 8 ) was assessed via a Mann–Whitney test. The P -value is ranked based on the exact value given by the software. All error bars show s.d. In one experiment, it was not possible to run any statistical test because of the nature of the data. To count ciliated cells in the tracheas of embryos, we had to compare individuals within the same litter to avoid bias arising from possible developmental differences between two litters. Consequently, there were too few embryos in each litter to perform statistical testing. FACS analysis Cell cycle profiles of cycling as well as serum-starved WT or Cyld Δ932 MEFs were determined by analysing total DNA content using propidium iodide staining (1 h incubation of ethanol-fixed cells in PBS containing 20 μg ml −1 propidium iodide, 100 μg ml −1 RNase A, and 0.1% Triton X-100). Cells were subjected to flow cytometry by using a FACSCalibur analyser (BD Biosciences) and the results were analysed with FlowJo. NF-κB inhibition by IκBα-SR RPE1 cells were transfected by GFP-PACT-CYLD WT , GFP-PACT-CYLD H/N or GFP-PACT-CYLD Δ932 plasmids in the presence of an Ig-κB-Luc reporter plasmid with or without a plasmid expressing a non-degradable form of IκBα (IκBα-SR) [41] . Cells were serum starved 24 h after transfection to induce cilia formation and fixed 48 h after serum depletion for cilia analysis. To measure the effect of IκBα-SR, cells were stimulated with 10 ng ml −1 of TNF-α just before removing the serum (24 h after transfection) or 3 h before completing the experiment. Cell extracts were prepared and Ig-κB-Luciferase-derived activity measured using a LB 9507 Berthold Luminometer. How to cite this article: Eguether, T. et al. The deubiquitinating enzyme CYLD controls apical docking of basal bodies in ciliated epithelial cells. Nat. Commun. 5:4585 doi: 10.1038/ncomms5585 (2014).